Probing transcription factor diffusion dynamics in the living mammalian embryo with photoactivatable fluorescence correlation spectroscopy Transcription factors use diffusion to search the DNA, yet the mechanisms controlling transcription factor diffusion during mammalian development remain poorly understood. Here we combine photoactivation and fluorescence correlation spectroscopy to study transcription factor diffusion in developing mouse embryos. We show that the pluripotency-associated transcription factor Oct4 displays both fast and Brownian and slower subdiffusive behaviours that are controlled by DNA interactions. Following cell lineage specification, the slower DNA-interacting diffusion fraction distinguishes pluripotent from extraembryonic cell nuclei. Similar to Oct4, Sox2 shows slower diffusion in pluripotent cells while Cdx2 displays opposite dynamics, suggesting that slow diffusion may represent a general feature of transcription factors in lineages where they are essential. Slow Oct4 subdiffusive behaviours are conserved in embryonic stem cells and induced pluripotent stem cells (iPS cells), and lost during differentiation. We also show that Oct4 diffusion depends on its interaction with ERG-associated protein with SET domain. Photoactivation and fluorescence correlation spectroscopy provides a new intravital approach to study transcription factor diffusion in complex in vivo systems. A complete understanding of the role of transcription factors (TFs) in controlling cell differentiation during development requires multi-level information about their dynamic features within the cell. Recent advances in single-cell imaging have made it possible to relate dynamic oscillations in the subcellular localization of TFs to changes in gene expression and cell fate in cultured cells [1] , [2] , [3] , [4] . Furthermore, we have recently shown that the rates of nucleocytoplasmic transport and nuclear retention of a TF are linked to cell lineage patterning in mouse embryos [5] . The basis of most TF biological functions, however, relies on their dynamic mobility and ability to interact with DNA inside the cell nucleus. Studies have shown that TFs are highly mobile inside mammalian cell nuclei [6] , and it is now clear that TFs use diffusion as the prime means of searching the genome [7] , [8] , [9] . Moreover, other proteins controlling DNA have been shown to change their diffusion properties during different cell behaviours including responses to extracellular signals [10] , [11] and DNA damage [12] . Together, these studies suggest that TF diffusion could be dynamically controlled by cell differentiation events occurring during embryogenesis. However, the diffusion properties of TFs controlling cell differentiation could not be investigated so far with current methods directly in developing mammalian organisms. Fluorescence correlation spectroscopy (FCS) is well suited for measurements of rapid protein diffusion at submicrometer scales [13] , [14] . This method has classically been applied to measure diffusion of molecules in solution, and more recently also the diffusion of proteins in the extracellular space of fish embryos [15] . Nevertheless, like most technologies based on fluorescence imaging, the combination of high concentrations of fluorescent molecules with high-energy illumination frequently causes photobleaching [14] , [16] , [17] . This phenomenon can lead to toxic chemical species and has largely prevented studies of protein diffusion in mammalian cells deep inside organisms, especially for proteins, such as TFs that are typically expressed at high levels [8] , [18] . Photobleaching has been minimized in culture conditions by selecting transfected cells that express minimal levels of labelled proteins [14] , [17] , using high-laser intensity to photobleach some of the initial fraction of fluorescent molecules [17] , or using heat-shock controllable promoters in Drosophila [19] . However, these approaches cannot be readily applied in developing mammalian embryos and ideally, FCS experiments should be independent of protein expression levels. Here, in order to non-invasively investigate TF diffusion properties in single-cell nuclei during mammalian development, we have combined FCS with the use of the photoactivatable green fluorescent protein (paGFP) [20] , which allowed us to control the number of fluorescently labelled TFs during measurements. We applied this new photoactivation and fluorescence correlation spectroscopy (paFCS) approach to reveal dynamic changes and the mechanisms controlling the diffusion of Oct4, a TF critical for pluripotency [21] , [22] during cell differentiation in developing mouse embryos and stem cells. Applying paFCS to quantify TF diffusion in living embryos The preimplantation mouse embryo initially comprises undifferentiated cells, which by blastocyst stage generate the first distinguishable cell lineages [23] , [24] . To measure TF diffusion in embryos, we first microinjected into one-cell stage embryos RNA coding for a photoactivatable form of the TF Oct4 (Oct4-paGFP) with RNA coding for histone 2B fused to RFP (H2B-RFP) to visualize each cell nucleus. We have previously shown that Oct4-paGFP is expressed within the physiological range of the wild-type protein, and that it can be selectively photoactivated with 820 nm light in cell nuclei [5] ( Fig. 1a and Supplementary Fig. S1 ). We then determined the position of the H2B-RFP-labelled nuclei and performed one photoactivation iteration at a single Z position covering the nucleus ( Fig. 1a ). Immediately after photoactivation, excitation with 488 nm light revealed an increase in fluorescence above background levels ( Fig. 1b ). We then determined how increasing fluorescence by photoactivation reflected on the quality of paFCS data in two-cell embryos ( Fig. 1b ), a developmental stage that precedes the first outward signs of cell differentiation [23] , [24] . During these experiments, fluctuations in fluorescence intensity are recorded as molecules diffuse through a small detection volume and their dwell time ( τD ) and diffusion coefficient can be obtained from analysis of the autocorrelation function (ACF) curves ( Fig. 1a ). Applying one photoactivation iteration produced stable count rates ( Fig. 1c ) and satisfactory ACFs ( Fig. 1d ). However, while applying two or three photoactivation iterations increased the mean count rates, the amplitude of the ACFs decreased and the signal-to-noise (S/N) ratio deteriorated ( Fig. 1c ). The mean count rates in non-photoactivated nuclei were >10-fold lower than when applying photoactivation and this negligible background fluorescence (<10%) was uncorrelated ( Fig. 1d ). There was no increase in mean count rates during measurements performed in non-photoactivated nuclei, indicating that the excitation light did not cause photoactivation during measurement ( Fig. 1c ). To rule-out the possibility that geometry or timing of photoactivation affected the diffusion behaviours, we compared ACFs from nuclei photoactivated at three different Z positions with one-third of the laser intensity ( Supplementary Fig. S2 ), and ACFs obtained 3 min or 2 h after photoactivation ( Supplementary Fig. S2 ). The ACFs from these experiments were indistinguishable. Moreover, we obtained similar ACFs with different Oct4-paGFP RNA concentrations ( Supplementary Fig. S3 ). Together, these experiments show that tuning the number of fluorescent species by photoactivation permits ready optimization of the quality of paFCS experiments in developing embryos. 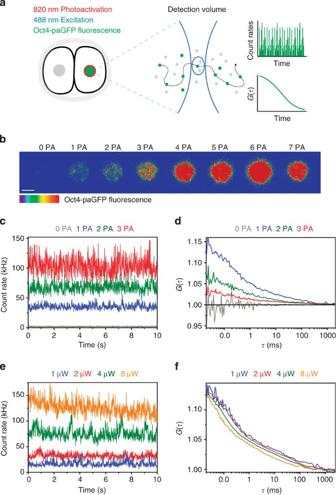Figure 1: paFCS permits tunability of Oct4-paGFP fluorescence (a) Single-cell nuclei of the embryo are selectively photoactivated with 820 nm light. A low number of photoactivated Oct4-paGFP molecules diffuse through the detection volume and are excited by 488 nm light. Fluctuations in fluorescence are used to generate the ACF (G(τ)) and reveal Oct4-paGFP diffusion properties. (b) Cell nucleus of a live embryo expressing Oct4-paGFP showing fluorescence intensity following multiple photoactivation (PA) iterations. Scale bar, 10 μm. (c,d) Count rates recorded over time in the same cell nucleus (c) following 0, 1, 2 and 3 photoactivation iterations with corresponding ACFs (d). The ACF resulting from one photoactivation iteration displays the most optimized amplitude and signal-to-noise. (e,f) Count rates recorded over time (e) in the same cell nucleus with increasing 488 nm laser intensities (from ~1 to 8 μW measured at back aperture of the objective) with their corresponding ACFs (f). At laser intensities of ~1 and ~2 μW fluorescence intensity traces were stable and ACFs were similar. Figure 1: paFCS permits tunability of Oct4-paGFP fluorescence ( a ) Single-cell nuclei of the embryo are selectively photoactivated with 820 nm light. A low number of photoactivated Oct4-paGFP molecules diffuse through the detection volume and are excited by 488 nm light. Fluctuations in fluorescence are used to generate the ACF (G( τ )) and reveal Oct4-paGFP diffusion properties. ( b ) Cell nucleus of a live embryo expressing Oct4-paGFP showing fluorescence intensity following multiple photoactivation (PA) iterations. Scale bar, 10 μm. ( c , d ) Count rates recorded over time in the same cell nucleus ( c ) following 0, 1, 2 and 3 photoactivation iterations with corresponding ACFs ( d ). The ACF resulting from one photoactivation iteration displays the most optimized amplitude and signal-to-noise. ( e , f ) Count rates recorded over time ( e ) in the same cell nucleus with increasing 488 nm laser intensities (from ~1 to 8 μW measured at back aperture of the objective) with their corresponding ACFs ( f ). At laser intensities of ~1 and ~2 μW fluorescence intensity traces were stable and ACFs were similar. Full size image To assess whether photobleaching could affect the diffusion behaviours observed, we performed consecutive measurements of fluorescence fluctuations within the same detection volume of a single photoactivated nucleus with different laser intensities. At laser intensities of ~1 and ~2 μW the fluorescence intensity traces were stable and the ACFs and diffusion parameters were similar ( Fig. 1e ). Moreover, no significant decrease in mean count rates was observed over the duration of typical Oct4-paGFP measurements ( Supplementary Fig. S4 ). However, increasing laser intensity to ~4 μW caused a left-shift of the ACF and a decrease in dwell time values, leading to an apparently faster Oct4-paGFP diffusion behaviour ( Fig. 1f ). At ~8 μW these effects were more pronounced and photobleaching was visible with a decay of mean count rates ( Fig. 1e ). We thus performed our experiments using ~1–~2 μW. Oct4-paGFP displays Brownian and anomalous diffusion To gain information about Oct4-paGFP diffusion properties, the ACFs generated for Oct4-paGFP in two-cell embryos ( Fig. 2a ) were fitted to appropriate models ( Fig. 2c–f ). The simplest model comprising a term to account for triplet state photophysics and a 3-dimensional Brownian (random) diffusion component provided unsatisfactory fitting. Adding a second diffusion component improved the fitting and implied the existence of two diffusion components, yet the model did not fit the slower component satisfactorily. This suggested that the diffusion of the slower molecules may be altered and prompted us to test a two-component model in which the second component accounts for anomalous subdiffusive processes. This empirical model provided satisfactory fitting and allowed us to quantitatively describe Oct4-paGFP diffusion properties ( Fig. 2g–i and Table 1 ). 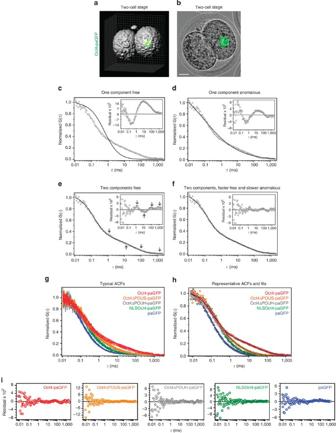Figure 2: Oct4-paGFP diffusion properties in living two-cell mouse embryos. (a,b) Three-dimensional surface rendered (a) and single plane (b) images of a two-cell embryo showing Oct4-paGFP fluorescence in one photoactivated cell nucleus. (c–f) Comparison of different fitting models for Oct4-paGFP. Models with one free component (c), one anomalous component (d) and two free components (e) did not provide satisfactory fits to the ACF. A satisfactory fit was obtained with a two-component model with the faster component being free and the slower component being anomalous (f), and was used to fit all ACFs in this study. Arrows ineindicate regions of poor fit of the model with two free components to the ACF. Smaller graphs show fit residuals. (g,h) Typical ACFs from at least 10 cells (g) with a representative ACF and fit results (h) for each protein measured by paFCS at the two-cell stage. While Oct4-paGFP (red) displays a two-component diffusion behaviour with a freely diffusing fraction and a slower fraction diffusing anomalously, the slower fraction is faster when the DNA-binding domains in Oct4ΔPOUS-paGFP (orange) and Oct4ΔPOUH-paGFP (grey) are truncated. paGFP (blue) and NLSOct4-paGFP (green) display essentially Brownian diffusion. (i) Individual fit residuals for data shown inh. Scale bar, 15 μm. Figure 2: Oct4-paGFP diffusion properties in living two-cell mouse embryos. ( a , b ) Three-dimensional surface rendered ( a ) and single plane ( b ) images of a two-cell embryo showing Oct4-paGFP fluorescence in one photoactivated cell nucleus. ( c – f ) Comparison of different fitting models for Oct4-paGFP. Models with one free component ( c ), one anomalous component ( d ) and two free components ( e ) did not provide satisfactory fits to the ACF. A satisfactory fit was obtained with a two-component model with the faster component being free and the slower component being anomalous ( f ), and was used to fit all ACFs in this study. Arrows in e indicate regions of poor fit of the model with two free components to the ACF. Smaller graphs show fit residuals. ( g , h ) Typical ACFs from at least 10 cells ( g ) with a representative ACF and fit results ( h ) for each protein measured by paFCS at the two-cell stage. While Oct4-paGFP (red) displays a two-component diffusion behaviour with a freely diffusing fraction and a slower fraction diffusing anomalously, the slower fraction is faster when the DNA-binding domains in Oct4ΔPOU S -paGFP (orange) and Oct4ΔPOU H -paGFP (grey) are truncated. paGFP (blue) and NLS Oct4 -paGFP (green) display essentially Brownian diffusion. ( i ) Individual fit residuals for data shown in h . Scale bar, 15 μm. Full size image Table 1 Summary of diffusion parameters in embryos. Full size table The faster Oct4-paGFP diffusion component represented 75% of the molecules and showed dwell times in the range of 120–220 μs. From these dwell times, we calculated the average diffusion coefficient to be D free =52.6±1.6 μm 2 s −1 . The second Oct4-paGFP component represented ~25% of the molecules, showed dwell times in the order of tens of milliseconds and anomaly parameters α slow significantly lower than 1 ( α slow <1 indicates anomalous behaviour). The average anomaly parameter ( α slow =0.73) and dwell time ( τD slow =13.4 ms) yielded a transport coefficient Γ slow /4 of 1.34±0.11 μm 2 s −1 (see Methods for transport coefficient [25] ). A reaction-dominant model [26] applied to chromatin-binding proteins, where one component accounts for free diffusion and the other contains rate constants for binding and unbinding to DNA, did not provide satisfactory fitting, implying that the slower component cannot be described solely by a binding reaction ( Supplementary Fig. S5 ). We also cannot exclude the existence of a small pool of immobile TFs. To further validate our approach, we compared our results to those obtained using Oct4 tagged with GFP (Oct4-GFP). We applied a prebleaching step, which is typically needed to reduce the initial concentration of fluorescent molecules [17] . While prebleaching nuclei compromised cell viability and was unsuitable for non-invasive work in living embryos, we could apply this approach in cultured embryonic stem (ES) cells, where Oct4-GFP displayed free and slower diffusion components similarly to Oct4-paGFP in embryos ( Supplementary Fig. S6 ). Slow Oct4-paGFP diffusion is controlled by DNA interactions To further characterize the two Oct4-paGFP components, we first determined whether the faster component reflects freely diffusing molecules by comparison with paGFP alone ( Fig. 2g–i and Table 1 ). As expected, the ACFs for paGFP showed that the majority of molecules (89%) diffuse freely ( D free =65.7±2.6 μm 2 s −1 ). The remaining 11% was accounted for by the second slower component, yet unlike the slower component of Oct4-paGFP, that of paGFP was essentially non-anomalous. A paGFP fusion protein tagged at its amino-terminal region by the putative nuclear localization signal (NLS) of Oct4 [27] (NLS Oct4 -paGFP) showed similar diffusion behaviour to paGFP ( D free =49.9±4.3 μm 2 s −1 , 87%) ( Fig. 2g–l and Table 1 ). The slightly slower free diffusion of NLS Oct4 -paGFP compared with paGFP likely results from interactions between the NLS and transport machinery [28] . The reduction in the free diffusion coefficient is consistent with differences in molecular weight (66 kDa for Oct4-paGFP and 27 kDa for paGFP) [13] . The dwell time and anomaly parameters of the slower Oct4-paGFP component indicate that these molecules undergo interactions that slow their mobility and imply that their diffusion is no longer Brownian. Anomaly parameters less than one indicate subdiffusive or hindered behaviour [29] . To investigate whether this behaviour could result from interactions with DNA, we measured the diffusion of a modified protein in which the POU-specific domain (POU S ) of Oct4, which is necessary for DNA binding [30] , [31] , was truncated (Oct4ΔPOU S -paGFP). Oct4ΔPOU S -paGFP showed a freely diffusing component accounting for 72% of molecules ( D free =42.9±1.5 μm 2 s −1 ). However, the behaviour of the slower component was both faster (Γ slow /4=1.96±0.24 μm 2 s −1 ) and less anomalous ( α slow =0.93) than the slower component of Oct4-paGFP ( Fig. 2g–i and Table 1 ). This finding was supported by performing paFCS measurements on another truncated version of Oct4 in which the homeodomain-specific region of the POU domain (POU H ), which cooperates with the POU S region to bind DNA [31] , was deleted. Oct4ΔPOU H -paGFP displayed similar diffusion behaviour to Oct4ΔPOU S -paGFP ( Fig. 2g–i and Table 1 ). Furthermore, we also investigated a protein carrying a single point mutation affecting Oct4's DNA-binding ability but intact transactivation domains [32] (Oct4 V234P -paGFP), which displayed similar diffusion properties to those observed with the POU S and POU H truncations ( Supplementary Fig. S7 ). Moreover, as was the case for the truncated proteins, microinjection of short double-stranded oligonucleotides containing consensus Oct4-DNA-binding sites [33] resulted in the slower fraction of Oct4-paGFP displaying faster and less anomalous diffusion ( Supplementary Fig. S8 ). Together, these results indicate that DNA interactions control the diffusion of the slower fraction of Oct4-paGFP in the embryo. Cell lineage specification leads to changes in TF diffusion We have previously shown that differences in Oct4-paGFP nucleocytoplasmic transport and nuclear retention distinguish the first cell lineages of the embryo [5] : the trophectoderm that contributes to extraembryonic structures, and the pluripotent inner cell mass (ICM) that gives rise to the foetus [23] , [24] . Our previous work suggested the existence of differences at the intranuclear level in the nature of Oct4-DNA interactions between these lineages [5] , [34] , yet it remained difficult to obtain information relating the biophysical properties of TFs to intranuclear differences between lineages. Thus, we then asked whether lineage specification could be revealed by the diffusion properties of TFs in the early blastocyst, a developmental stage by which cells have been allocated to their inside (pluripotent) and outside (extraembryonic) positions within the embryo ( Fig. 3a ). In both lineages, ACFs were similar to those obtained at the two-cell stage and required a model with one component diffusing freely, and another component diffusing slowly and anomalously ( Fig. 3c–e and Table 1 ). The slower component displayed anomalous behaviour and fractions that were similar to those measured at the two-cell stage. However, while in extraembryonic cells the dwell time of the slower component ( τD slow of 11.0 ms) was similar to that measured at the two-cell stage, in pluripotent cells ( τD slow of 48.0 ms) it was 4.3-fold larger ( Table 1 ). The diffusion coefficient of the free component was reduced by 1.6-fold in pluripotent cells compared with the two-cell stage and it remained unchanged in extraembryonic cells, suggesting that different factors control the free fraction by this stage ( Table 1 ). paGFP diffusion properties in the two lineages were similar to the two-cell stage, indicating that the differences in Oct4-paGFP diffusion are specific to the TF and unlikely to result from changes in cellular viscosity ( Table 1 and Supplementary Fig. S9 ). These findings thus show that during preimplantation development, the diffusion properties of Oct4-paGFP become slower in the pluripotent cell lineage in which Oct4 functions are essential [21] , [22] , and faster in cells committed to extraembryonic structures. 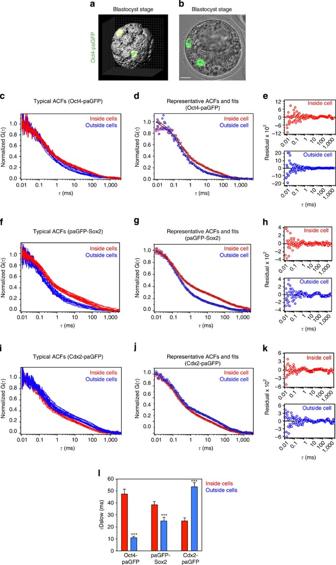Figure 3: TF diffusion properties identify cell lineages of the blastocyst. (a,b) Three-dimensional surface rendered (a) and single plane (b) images of a blastocyst stage embryo showing Oct4-paGFP fluorescence in the photoactivated nuclei of a pluripotent cell deep within the inside region of the embryo (bottom cell) and an extraembryonic cell within the outside region of the embryo (upper cell). (c,d,f,g,i,j) Typical ACFs from at least 10 cells (c) with a representative ACF and fit results (d) for Oct4-paGFP in pluripotent and extraembryonic cells. Oct4-paGFP displays slower diffusion in the pluripotent cell. (e) Fit residuals for data shown ind. (f,g) Typical ACFs from at least 10 cells (f) with a representative ACF and fit results (g) for paGFP-Sox2 in inside and outside cells. paGFP-Sox2 displays slower diffusion behaviours in inside cells. (i,j) Typical ACFs from at least 10 cells (i) with a representative ACF and fit results (j) for Cdx2-paGFP in inside and outside cells. Cdx2-paGFP displays slower diffusion behaviours in outside cells. (h,k) Fit residuals for data shown ing,j. (l) Bar charts of mean±s.e. ofτDslowfor Oct4-paGFP (n≥36), paGFP-Sox2 (n≥24) and Cdx2-paGFP (n≥15) in inside and outside cells; see alsoTable 1(***P<0.0001; Student’st-test). Scale bars, 15 μm. Figure 3: TF diffusion properties identify cell lineages of the blastocyst. ( a , b ) Three-dimensional surface rendered ( a ) and single plane ( b ) images of a blastocyst stage embryo showing Oct4-paGFP fluorescence in the photoactivated nuclei of a pluripotent cell deep within the inside region of the embryo (bottom cell) and an extraembryonic cell within the outside region of the embryo (upper cell). ( c , d , f , g , i , j ) Typical ACFs from at least 10 cells ( c ) with a representative ACF and fit results ( d ) for Oct4-paGFP in pluripotent and extraembryonic cells. Oct4-paGFP displays slower diffusion in the pluripotent cell. ( e ) Fit residuals for data shown in d . ( f,g ) Typical ACFs from at least 10 cells ( f ) with a representative ACF and fit results ( g ) for paGFP-Sox2 in inside and outside cells. paGFP-Sox2 displays slower diffusion behaviours in inside cells. ( i,j ) Typical ACFs from at least 10 cells ( i ) with a representative ACF and fit results ( j ) for Cdx2-paGFP in inside and outside cells. Cdx2-paGFP displays slower diffusion behaviours in outside cells. ( h,k ) Fit residuals for data shown in g,j . ( l ) Bar charts of mean±s.e. of τD slow for Oct4-paGFP ( n ≥36), paGFP-Sox2 ( n ≥24) and Cdx2-paGFP ( n ≥15) in inside and outside cells; see also Table 1 (*** P <0.0001; Student’s t -test). Scale bars, 15 μm. Full size image Similarly to Oct4, Sox2 functions have classically been associated with pluripotency [35] , while Cdx2 functions have been linked to the specification of extraembryonic cells [36] . By early blastocyst stage, Sox2 and Cdx2 are expressed in both inside and outside cells of the embryo, albeit their expression levels are often heterogeneous [23] , [24] , [36] . Similarly to Oct4-paGFP, paFCS measurements of paGFP-Sox2 and Cdx2-paGFP produced ACFs fitting to a two-component model with the slower diffusion component being anomalous ( Fig. 3f–k and Table 1 ). However, while the slower diffusion component of paGFP-Sox2 displayed larger dwell times in inside cells ( τD slow of 39.0 ms) compared with outside cells ( τD slow of 29.0 ms) similarly to Oct4-paGFP, the slower diffusion component of Cdx2-paGFP displayed smaller dwell times in inside cells ( τD slow of 25.0 ms) compared with outside cells ( τD slow of 54.0 ms) ( Fig. 3l ). Thus, slower diffusion dynamics are a general feature of these TFs in the lineages where they are best known to have key functional roles. Oct4-paGFP diffusion is conserved in pluripotent cell types Pluripotent ES cell lines can be derived from mammalian embryos, yet it remains unclear to what extent they share properties with pluripotent cells in their native embryonic environment [37] . Thus, we next investigated whether ES cells share similar Oct4-paGFP diffusion properties with their in vivo counterparts. As was the case in the embryo, the ACFs required a two-component diffusion model for fitting ( Fig. 4a–h and Table 2 ). The slower component displayed anomalous behaviour (Γ slow /4=0.34±0.03 μm 2 s −1 α slow =0.87), while the faster component displayed free diffusion ( D free =41.0±1.1 μm 2 s −1 ). Furthermore, the Oct4ΔPOU S -paGFP and Oct4ΔPOU H -paGFP proteins displayed smaller dwell times of their slower fraction compared with Oct4-paGFP ( Fig. 4b and Table 2 ). Thus, Oct4-paGFP diffusion properties in ES cells mirror those found in pluripotent cells of the embryo. 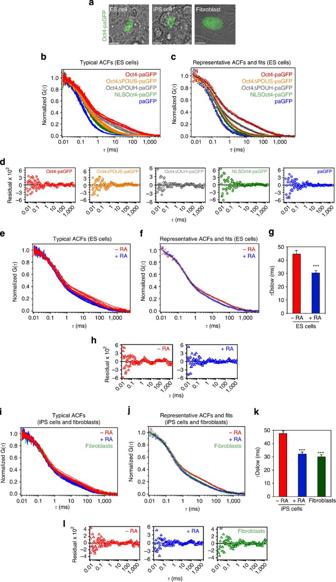Figure 4: Oct4-paGFP diffusion properties in ES cells and iPS cells. (a) Images show Oct4-paGFP fluorescence in a single photoactivated nucleus of an ES cell, iPS cell and fibroblast cell. (b,c,e,f,i,j) Typical ACFs from at least 10 cells (b,e,i) with corresponding representative ACFs, fit results (c,f,j) and fit residuals (d,h,l). Oct4-paGFP (red) in ES cells (b,c,e,f) and iPS cells (i,j) displays a two-component diffusion behaviour similar to pluripotent cells in blastocyst stage embryos, with a freely diffusing and a slower and anomalous fraction. Oct4ΔPOUS-paGFP (orange), Oct4ΔPOUH-paGFP (grey), NLSOct4-paGFP (green) and paGFP (blue) display similar diffusion behaviours as in two-cell embryos (b–d). Treatment with retinoic acid (RA) causes changes in the mean dwell times of the Oct4-paGFP slower component in ES cells (e–h) and in iPS cells (i–l), which resemble the dwell times measured in fibroblasts. (g,k) Bar charts of mean±s.e. ofτDslowfor Oct4-paGFP in ES cells (n≥20) (g), iPS cells (n≥20) and fibroblasts (n=14) (k); see alsoTable 2(***P<0.0001; Student’st-test). Scale bars, 15 μm. Figure 4: Oct4-paGFP diffusion properties in ES cells and iPS cells. ( a ) Images show Oct4-paGFP fluorescence in a single photoactivated nucleus of an ES cell, iPS cell and fibroblast cell. ( b , c , e , f , i , j ) Typical ACFs from at least 10 cells ( b , e , i ) with corresponding representative ACFs, fit results ( c , f , j ) and fit residuals ( d , h , l ). Oct4-paGFP (red) in ES cells ( b , c , e , f ) and iPS cells ( i , j ) displays a two-component diffusion behaviour similar to pluripotent cells in blastocyst stage embryos, with a freely diffusing and a slower and anomalous fraction. Oct4ΔPOU S -paGFP (orange), Oct4ΔPOU H -paGFP (grey), NLS Oct4 -paGFP (green) and paGFP (blue) display similar diffusion behaviours as in two-cell embryos ( b – d ). Treatment with retinoic acid (RA) causes changes in the mean dwell times of the Oct4-paGFP slower component in ES cells ( e – h ) and in iPS cells ( i – l ), which resemble the dwell times measured in fibroblasts. ( g , k ) Bar charts of mean±s.e. of τD slow for Oct4-paGFP in ES cells ( n ≥20) ( g ), iPS cells ( n ≥20) and fibroblasts ( n =14) ( k ); see also Table 2 (*** P <0.0001; Student’s t -test). Scale bars, 15 μm. Full size image Table 2 Summary of Oct4-paGFP diffusion parameters in ES cells and iPS cells. Full size table We next asked whether Oct4-paGFP diffusion properties would also be shared by iPS cells obtained by reprogramming somatic cell types. Measuring Oct4-paGFP diffusion in iPS cells derived from fibroblasts produced ACFs and diffusion parameters similar to those obtained in ES cells and in the pluripotent cells of the embryo ( Fig. 4i–l and Table 2 ). The slower component again displayed anomalous behaviour (Γ slow /4=0.32±0.04 μm 2 s −1 , α slow =0.87), while the faster component displayed free diffusion ( D free =39.1±1.0 μm 2 s −1 ). Finally, we determined whether Oct4-paGFP diffusion could be modified when ES cells and iPS cells differentiate following treatment with retinoic acid. Significantly reduced dwell times of the slower Oct4-paGFP fraction were quantified after 48 h of treatment for both ES cells and iPS cells ( Fig. 4e–l and Table 2 ). Moreover, the diffusion properties measured following retinoic acid treatment were similar to those obtained for Oct4-paGFP in mouse embryonic fibroblasts ( Fig. 4i–l ). Together, these results indicate that distinct Oct4-paGFP diffusion properties are conserved across different pluripotent cell types. Interactions with ESET contribute to Oct4-paGFP diffusion We finally explored how chromatin states, post-translational modifications and interactions with other proteins, may impact on Oct4-paGFP diffusion. To test whether global chromatin manipulations affect TF diffusion we treated ES cells with Trichostatin A (TSA), which causes general chromatin decompaction [17] , [38] or Actinomycin D that induces chromatin compaction [17] , [39] . While TSA led to significantly larger dwell times, Actinomycin D led to smaller dwell times of the slower Oct4-paGFP diffusion component ( Supplementary Fig. S10 ). Neither TSA nor Actinomycin D caused changes in the diffusion of Oct4ΔPOU H -paGFP ( Supplementary Fig. 9 ), suggesting that global chromatin compaction can affect TF diffusion properties by changing DNA accessibility to the TF. Post-translational modification of Oct4 by SUMOylation has been shown to affect its transcriptional activities in different cellular systems [33] , [40] , [41] . However, a K118R point mutation impairing Oct4 SUMOylation by SUMO-1 ( [33] ) (Oct4 K118R -paGFP) resulted in essentially similar diffusion properties compared with Oct4-paGFP, and did not result in differentiated ES cell morphology 48 h post transfection ( Supplementary Fig. S11 ). This suggests that Oct4 SUMOylation does not control its diffusion properties, which is in agreement with apparently normal development of the pluripotent lineage in sumo1 -null embryos [42] . Finally, we determined whether interactions with other proteins involved in gene regulation might control Oct4-paGFP diffusion properties. The methyltransferase ERG-associated protein with SET domain (ESET) was recently identified as a binding partner of Oct4 important for pluripotency [43] , [44] . Interfering with ESET in embryos leads to failure of cells to integrate into the ICM and eset -null embryos [45] display defects in the pluripotent lineage, dying around implantation stages. To investigate whether ESET controls Oct4-paGFP diffusion properties, we microinjected ESET siRNAs into one cell of two-cell embryos and measured Oct4-paGFP diffusion properties at the eight-cell stage. This developmental stage precedes the internalization of cells to the inner regions of the compacted morula, which contribute to the pluripotent lineage [23] , [24] , [46] . In cells microinjected with a control small interfering RNA (siRNA), the ACFs required a two-component diffusion model for fitting, with a slower component displaying anomalous behaviour with a dwell time τD slow of 36.0 ms ( Fig. 5a–d and Table 1 ). By contrast, in cells microinjected with the ESET siRNA, Oct4-paGFP displayed significantly smaller dwell times with a τD slow of 16.0 ms ( Fig. 5a–d and Table 1 ). 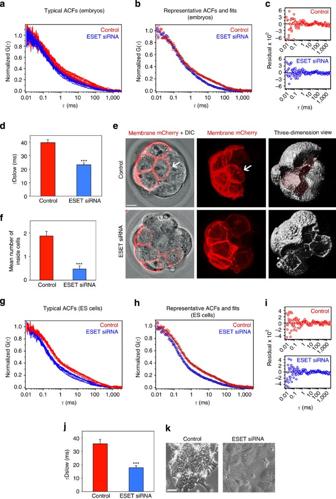Figure 5: ESET controls Oct4-paGFP diffusion properties. (a,b) Typical ACFs from at least 10 cells (a) with a representative ACF and fit results (b) for Oct4-paGFP in eight-cell stage embryos. The embryos were microinjected with control (red) or ESET siRNA (blue) in one cell at the two-cell stage. (c) Fit residuals for data shown inb. (d) Bar charts of mean±s.e. ofτDslowfor Oct4-paGFP at the two-cell stage reveal significantly smallerτDslowfor embryos microinjected with ESET siRNA compared with control siRNA; see alsoTable 1(n≥18). (e) Single plane images (left panel), three-dimensional reconstructions (middle panel) and three-dimensional surface renderings (right panel) were used to reveal the position of cells labelled with a membrane-targeted mCherry coinjected with ESET or control siRNA at the 16-cell stage. Embryos microinjected with the ESET siRNA exhibit fewer cells in the inside regions of the morula. The white arrow shows the typical position of a cell within the inside region of the morula in a control embryo. Two inside cells are clearly visible in the three-dimensional rendering (pseudo-labelled in pink) in the control embryo (right panel). (f) Bar chart of mean±s.e. of number of internalized inside cells (n=15 embryos). Significantly reduced numbers of inside cells were found in embryos injected with ESET siRNA, compared with the control by the 16-cell stage. (g,h) Typical ACFs from at least 10 cells (g) with a representative ACF and fit result (h) for Oct4-paGFP transfected in ES cells with 200 nM control or ESET siRNA. (i) Fit residuals for data shown inh. (j) Bar charts of mean±s.e. ofτDslowfor Oct4-paGFP reveal significantly smallerτDslowfor ES cells transfected with ESET siRNA compared with control siRNA; see alsoTable 2(n≥19). (k) Transfection of ESET siRNA resulted in a clear differentiated ES cell morphology 72 h post transfection. (***P<0.0001; Student’st-test). Scale bars, 15 μm. Figure 5: ESET controls Oct4-paGFP diffusion properties. ( a,b ) Typical ACFs from at least 10 cells ( a ) with a representative ACF and fit results ( b ) for Oct4-paGFP in eight-cell stage embryos. The embryos were microinjected with control (red) or ESET siRNA (blue) in one cell at the two-cell stage. ( c ) Fit residuals for data shown in b . ( d ) Bar charts of mean±s.e. of τD slow for Oct4-paGFP at the two-cell stage reveal significantly smaller τD slow for embryos microinjected with ESET siRNA compared with control siRNA; see also Table 1 ( n ≥18). ( e ) Single plane images (left panel), three-dimensional reconstructions (middle panel) and three-dimensional surface renderings (right panel) were used to reveal the position of cells labelled with a membrane-targeted mCherry coinjected with ESET or control siRNA at the 16-cell stage. Embryos microinjected with the ESET siRNA exhibit fewer cells in the inside regions of the morula. The white arrow shows the typical position of a cell within the inside region of the morula in a control embryo. Two inside cells are clearly visible in the three-dimensional rendering (pseudo-labelled in pink) in the control embryo (right panel). ( f ) Bar chart of mean±s.e. of number of internalized inside cells ( n =15 embryos). Significantly reduced numbers of inside cells were found in embryos injected with ESET siRNA, compared with the control by the 16-cell stage. ( g , h ) Typical ACFs from at least 10 cells ( g ) with a representative ACF and fit result ( h ) for Oct4-paGFP transfected in ES cells with 200 nM control or ESET siRNA. ( i ) Fit residuals for data shown in h . ( j ) Bar charts of mean±s.e. of τD slow for Oct4-paGFP reveal significantly smaller τD slow for ES cells transfected with ESET siRNA compared with control siRNA; see also Table 2 ( n ≥19). ( k ) Transfection of ESET siRNA resulted in a clear differentiated ES cell morphology 72 h post transfection. (*** P <0.0001; Student’s t -test). Scale bars, 15 μm. Full size image To determine how the differences in Oct4-paGFP diffusion between control and ESET siRNA-injected embryos might relate to cell lineage allocation, we coinjected RNA for a membrane-targeted mCherry protein at the two-cell stage, which allowed us to identify the positioning of cells in three-dimensional reconstructions of the embryos ( Fig. 5e ). By the 16-cell stage, the number of total cells was not affected by microinjection of the siRNA. In control embryos, we found on average 1.9±0.2 cells ( n =15 embryos) microinjected with the control siRNA within the inner regions of the morula, in agreement with previous work [46] . However, microinjection of ESET siRNA led to a reduced number of inside cells (0.5±0.1; n =15 embryos) ( Fig. 5e ). Thus, quantifiable changes in the diffusion properties of Oct4-paGFP in eight-cell embryos precede defects in the internalization of cells to the pluripotent lineage. Similarly to the situation in the embryo, 72 h following transfection of ESET siRNA into ES cells ( Fig. 5g–k and Supplementary Fig. S12 ) Oct4-paGFP displayed smaller dwell times of the slower component with a τD slow of 23.0 ms, compared with control siRNA ( τD slow of 40.0 ms) ( Fig. 5g–j ). Furthermore, ES cells transfected with the ESET siRNA exhibited a classic differentiated morphology, which is consistent with previous observations [43] , [44] ( Fig. 5k ). In agreement with the idea that ESET interactions control Oct4-paGFP diffusion properties, a protein carrying a mutation in the SUMOylation interacting domain (SIM) (Oct4ΔSIM-paGFP) required to interact with ESET, displayed smaller dwell times ( τD slow of 22.0 ms) and similarly to the effect of ESET siRNA, these cells also exhibited a differentiated morphology 48 h post transfection ( Supplementary Fig. S11 ). The ESET siRNA and SIM mutation also led to smaller dwell times of the free fraction of Oct4-paGFP, which suggests that part of the free fraction might interact with ESET independently of DNA binding in line with previous work [43] . Thus, our results in embryos and ES cells show that Oct4-paGFP diffusion properties depend not only on DNA interactions, but also on the TF's ability to interact with ESET. We have quantitatively described the diffusion properties of a TF in developing mouse embryos. paFCS allows non-invasive control over the concentration of fluorescent species independently of expression levels. By restricting the number of fluorescent species to values similar to those desired when applying FCS in solution [13] , this approach allowed us to obtain satisfactory ACFs in >90% of experiments. paFCS does not require a prebleach step. Moreover, the short time windows needed to obtain multiple ACFs makes this method ideal for collecting data from samples that are difficult to maintain under observation. As paFCS does not require custom-made microscopy systems it should also be applicable with other FCS modalities [47] , [48] , [49] . TF functions have recently been proposed to depend not only on expression levels, but also on dynamic changes in their localization within the cell [1] , [2] , [3] , [4] . Interestingly, while both pluripotent and extraembryonic cells of the early blastocyst express Oct4, knockout of the Oct4 gene ( pou5f1 ) affects predominantly the pluripotent lineage [22] . We previously observed higher retention of Oct4 in pluripotent compared with extraembryonic nuclei [5] , and hypothesized that although Oct4 is expressed in the two lineages, the cells may have intranuclear differences in Oct4 mobility related to DNA interactions [5] , [34] . The use of paFCS has now allowed us to reveal intranuclear differences related to TF-DNA interactions and demonstrate distinct diffusion dynamics in these lineages. We show that by blastocyst stage Oct4-paGFP shows changes in the diffusion dwell times of the DNA-interacting fraction, leading to slower diffusion in pluripotent and faster in extraembryonic nuclei. Moreover, paGFP-Sox2 displayed similar dynamics to Oct4-paGFP, while Cdx2 displayed opposite dynamics in pluripotent and extraembryonic nuclei, suggesting that slower diffusion properties may be a general feature of TFs in lineages where their functions are essential. This idea was further supported by our experiments in cultured cells. We show that ES cells and iPS cells share similar Oct4-paGFP diffusion properties with pluripotent cells in the embryo. Furthermore, the Oct4-paGFP slower diffusing component is modified upon stem cell differentiation, indicating that the slower fraction is a sensitive marker of pluripotent nuclei. These findings together show that lineage specification events central to development can lead to quantitative changes in the diffusion properties of TFs, even before the appearance of sharply segregated TF protein expression domains by late blastocyst stage [23] , [24] , [50] . The biophysical mechanisms by which TFs search the genome in organisms are not fully understood [7] , [8] , [9] . However, our findings provide in vivo support to early theoretical work [51] , [52] , [53] by showing that TF diffusion is more complex than random movement in solution. Oct4-paGFP displays not only rapid and Brownian, but also slower and anomalous subdiffusion behaviour. Our comparisons with freely diffusing proteins, Oct4 proteins bearing defective DNA-interacting domains and microinjection of synthetic oligonucleotides suggest that the slower subdiffusive component results from interactions between the POU domain and DNA [25] , [30] , [33] . Based on recent work in simpler experimental systems, it is feasible that the anomalous subdiffusion behaviour may comprise processes such as sliding, hopping and intersegmental transfer, which could reduce the dimensionality of movement [7] , [8] , [9] and increase the frequency of interactions with DNA in pluripotent nuclei. Finally, Oct4-paGFP diffusion also depends on interactions with the epigenetic regulator ESET. While ESET is expressed in both pluripotent and extraembryonic cells, its interaction with Oct4 has been associated with pluripotency and repression of extraembryonic genes [44] . It is possible that the diffusion of Oct4 is linked not only to the increased molecular weight of the Oct4-ESET complex, but also to the enzymatic activity of ESET [43] , [44] . Changing Oct4-paGFP diffusion by interfering with ESET may have some deterministic role in cell differentiation, as we established an association between smaller dwell times of the DNA-interacting component and a non-pluripotent, differentiated cellular state. Both ESET knockdown and mutating Oct4’s SIM domain led to faster diffusion of the slower component and caused ES cell differentiation. Moreover, ESET knockdown in embryos led to smaller dwell times of the slower component preceding defects in cell internalization to the pluripotent regions of the morula. In sum, because paFCS can reveal a quantifiable hallmark of pluripotent nuclei, it may help to monitor cell reprogramming. paFCS also provides a new approach for studying the interplay between patterning events and the diffusion of gene-regulatory molecules. Imaging and FCS measurements Embryos and stem cells were imaged using a Zeiss LSM 780 laser scanning confocal microscope and avalanche photodiodes of the Confocor 3 (Zeiss, Jena). Cell nuclei were identified by H2B-RFP expression. A water UV-VIS-IR C-Apochromat × 40 1.2 NA objective (Zeiss, Jena) was used for imaging, photoactivation and FCS. Fusion proteins containing paGFP were excited using 488 nm, and RFP using 561 nm laser lines. Emitted light was collected using the same objective and directed to detectors through appropriate filters to eliminate scattered excitation light. Multiphoton-based photoactivation was carried out following previously described protocols [5] using 820 nm light (~6 mW as measured at back aperture of the objective) from a Chameleon Vision laser (Coherent). Both 820 nm and 405 nm (~22 μW) could be successfully applied for photoactivation in cultured cells, leading to similar diffusion behaviours. We used the 820 nm for embryos, as it allowed targeting of specific regions along the Z axis, and 405 nm for cultured cells as the cells are flatter against the plastic dish. For experiments using Oct4-GFP, a prebleach step was performed homogeneously in the whole nucleus of ES cells using high-intensity 488 nm light (200–400 μW), in order to decrease fluorescence and obtain count rates similar to those used for measurements of Oct4-paGFP. Similar prebleach experiments were performed in embryos, but the prebleach step compromised the viability of the bleached cell. Pinhole alignments for 488 nm and 561 nm lasers were carried out following the Confocor 3 (Zeiss, Jena) guidelines and its size set to 1 airy unit. FCS measurements were performed inside photoactivated nuclei in regions homogenously labelled by H2B-RFP avoiding the nuclear envelope, nucleoli and regions of highly condensed H2B-RFP, which likely represent silenced heterochromatin [54] . We did not perform experiments in G1 nuclei, which can be identified by their smaller size compared with nuclei in the S/G2 phase. We also excluded cells that have already engaged in mitosis as the M-phase can also be identified by the compaction of the chromatin labelled with a fluorescently tagged H2B construct, as demonstrated by others [55] , [56] . Fluorescence intensity was recorded in 200 ns bins for 10–20 s with 7–10 repetitions. We monitored the integrity of the cell nucleus by measuring the average fluorescence intensities of paGFP and H2B-RFP in the whole nucleus before and post FCS measurement to rule-out any photobleaching effects during the measurement. FCS experiments during which the embryo moved as assessed in images taken prior and post measurements were excluded. FCS measurements in stem cells were performed with the same settings used for the embryos. Analysis of cell position following siRNA microinjection To determine cell positions in 16-cell embryos we acquired Z stacks of embryos microinjected with siRNAs and membrane-targetted mCherry RNA (30 ng μl −1 ). As only one cell of these embryos was microinjected at the two-cell stage, half of the cells showed mCherry labelling. Imaris Software (Bitplane) was used to obtain three-dimensional views. We determined whether labelled cells were allocated to outer or inner regions of the morula following previous criteria [5] , [24] , [46] . Outer cells have a large region of their membrane exposed to the zona pellucida surrounding the embryo, while inner cells are almost completely buried within the embryo and have no surface exposed to the zona pellucida. We confirmed the position of cells by adding and removing the bright field channel to determine the contour of the entire embryo and visualize the zona pellucida (not shown). We determined that in 16-cell embryos, on average two-labelled cells are located in inner regions, in line with recent reports [24] , [46] . FCS analysis The ACF G( τ ) of the fluorescence intensity for each 10 or 20 s measurement was calculated using the ZEN Software FCS modules (Zeiss, Jena). This function compares the fluorescence intensity at time t , I( t ), with that at a time shifted by an amount τ (the lagtime), I(t+ τ ) as a function of τ , that is, where the angled brackets indicate time-averaged values. A mean ACF for analysis was generated by averaging the 7–10 repeat measurements. On occasion, a very-large slow moving fluorescent object would pass through the detection volume leading to a long (seconds or more) fluctuation in the intensity and distortion of the ACF. When this occurred, the affected ACF was excluded from the data set. Only ~1 in 20 ACFs recorded in embryos and ~1 in 40 recorded in ES cells were excluded. Mean ACFs were fitted using the ZEN Software (Zeiss, Jena) using a model that comprised two three-dimensional diffusion terms, one free and one anomalous, and another term to account for triplet state photophysics: In this expression, N is the number of diffusing molecules, T is the triplet state fraction and τ T is the triplet state lifetime, f i is the fraction of each diffusing component and τD i its dwell time. T is normalised to the total of the fractions of the diffusing components which sum to 1. S is a structural parameter relating the dimensions of the confocal volume and is equal to ω z / ω r where ω z and ω r are the axial and radial extensions to 1/ e 2 of the confocal volume, which is approximately ellipsoidal in shape. α i is an anomaly parameter for each diffusing species that measures the deviation from Brownian or free diffusion which is the case when α =1. The diffusion is termed super-diffusion when α >1 and subdiffusion for α <1. Subdiffusion is also referred to as hindered diffusion and indicates that the displacement with time of the diffusing species is less than the mean square displacement characteristic of Brownian diffusion [9] . The diffusion coefficient for a species can be calculated from its dwell time and the radial dimension, ω r of the confocal volume, When the diffusion of a species is anomalous, a transport coefficient can be calculated using the dwell time and the anomaly parameter [25] , and the diffusion coefficient is now time-dependant and related to Γ i via, Thus when the diffusion is Brownian, Γ i =4 D i . The values of ω r and S were determined by measurement of ~1 nM solution of Atto488 in water at 25 °C, a highly photostable small molecule with a well-known diffusion coefficient of 400 μm 2 s −1 and very low triplet yield. The data were fitted by a single free diffusion component and returned values of 0.18 μm for ω r and 5.5 for S . The confocal volume dimensions were confirmed through measurement of GFP in KSOM+AA (Sigma) buffer, which was well fit to a single diffusion component plus triplet term and returned diffusion coefficients of 96.5±0.7 μm 2 s −1 ( n =4) and 111.0±1.0 μm 2 s −1 ( n =4) at 25 °C and 37 °C, respectively. These values are in agreement with other reports [57] and consistent with a 27-kDa protein under these conditions [57] . The fitting model was determined by starting with one non-anomalous diffusion component plus the triplet term, and adding diffusion components and/or anomaly parameters until fitting proved satisfactory. Goodness of fit was judged by examination of the residuals (data minus fit), which should be randomly distributed about zero and by the value of the reduced χ 2 parameter returned by the ZEN Software. The triplet term was allowed to be free (both time constant and magnitude) and returned values indicating that triplet lifetimes are of the order of microseconds and thus has little contribution to the ACF for lag values >0.01 ms. Free diffusion dwell times were typically >0.1 ms and slow diffusion >1 ms. This temporal segregation of triplet photophysics and diffusion phenomena is advantageous for robust and reliable fitting of ACFs. We used this model for all samples and it is in line with approaches taken by others [12] to fitting FCS data for TFs interacting with DNA. The rationale for using a two-component approach is that not all TFs are bound to DNA at all times and, therefore, there will be both unbound (‘freely’ diffusing) and bound (DNA interacting and assumed to be immobile) populations. Recent work [26] has applied a ‘diffusion and binding’ model where rate constants for association of the TF with DNA and for dissociation of the TF-DNA ‘complex’ are explicitly defined. The reaction-dominant model did not fit our data satisfactorily ( Supplementary Fig. S5 ). Therefore, we chose to analyse all our data using a traditional two-component approach with the addition that the slower component was allowed to be anomalous, to provide an empirical measure of the extent of deviation from Brownian diffusion of the slower component to compare across the range of samples and conditions studied. Also, anomalous diffusion has been observed in a wide range of experimental systems including live cells and the anomaly parameter can take into account (or reasonably model) a range of phenomena without needing a priori knowledge or make any assumptions regarding them [12] , [29] , [58] . Statistical analysis All statistical analyses were performed with GraphPad Prism 5 software using an unpaired, two-tailed Student’s t -test, with data presented as mean±s.e. How to cite this article: Kaur, G. et al . Probing transcription factor diffusion dynamics in the living mammalian embryo with photoactivatable fluorescence correlation spectroscopy. Nat. Commun. 4:1637 doi: 10.1038/ncomms2657 (2013).